A sodium-ion sulfide solid electrolyte with unprecedented conductivity at room temperature Solid electrolytes are key materials to enable solid-state rechargeable batteries, a promising technology that could address the safety and energy density issues. Here, we report a sulfide sodium-ion conductor, Na 2.88 Sb 0.88 W 0.12 S 4 , with conductivity superior to that of the benchmark electrolyte, Li 10 GeP 2 S 12 . Partial substitution of antimony in Na 3 SbS 4 with tungsten introduces sodium vacancies and tetragonal to cubic phase transition, giving rise to the highest room-temperature conductivity of 32 mS cm −1 for a sintered body, Na 2.88 Sb 0.88 W 0.12 S 4 . Moreover, this sulfide possesses additional advantages including stability against humid atmosphere and densification at much lower sintering temperatures than those (>1000 °C) of typical oxide sodium-ion conductors. The discovery of the fast sodium-ion conductors boosts the ongoing research for solid-state rechargeable battery technology with high safety, cost-effectiveness, large energy and power densities. Development of all-solid-state rechargeable batteries has been desired because they have superior characteristics, such as a long cycle life, high safety, high-energy density, and high rate capability [1] , [2] , [3] , [4] . To realize bulk-type solid-state batteries using electrodes and electrolyte particles, superior solid electrolytes with high ionic conductivity and good ductility are desired, as they can facilitate wide contact areas with active materials simply upon pressing, without a high-temperature-sintering process [5] . Sulfide solid electrolytes meet this demand. Among solid electrolytes, Li 10 GeP 2 S 12 (LGPS)-type crystalline sulfides [4] , [6] show excellent Li-ion conductivity of over 10 −2 S cm −1 , which is higher than that of the conventional organic liquid electrolyte used in lithium-ion batteries, considering its low Li + transference number (below 0.5). Since our discovery of cubic Na 3 PS 4 with a relatively high Na ion conductivity of >10 −4 S cm −1 in 2012 [7] , studies for developing new Na-ion-conducting sulfides [8] , [9] , [10] , [11] , [12] , [13] , [14] , [15] , [16] , [17] , [18] , [19] , [20] , [21] , [22] have rapidly increased. In 2016, a good Na-ion conductivity of 1 × 10 −3 S cm −1 was achieved in Na 2.9375 PS 3.9375 Cl 0.0625 [10] with Na vacancies and sodium antimony sulfide, Na 3 SbS 4 [11] , [12] , [13] . In addition, several other sulfides including Na 11 Sn 2 PS 12 [16] , [17] and Na 3 SbSe 4 [18] exhibit Na-ion conductivities higher than 10 −3 S cm −1 at 25 °C. However, Na 10 GeP 2 S 12 (NGPS) [22] exhibits a moderate Na-ion conductivity of 10 −5 S cm −1 , which is much lower than the Li-ion conductivity of LGPS, implying that compositions that impart good Li-ion conductivity do not essentially impart good Na-ion conductivity. Further, typical oxide crystalline electrolytes of NASICON [23] and β -alumina [24] sintered at high temperatures show a high Na-ion conductivity of 10 −3 S cm −1 . As for electrolytes with typical NASICON structure, the Na-ion conductivity in Na 3 Zr 2 Si 2 PO 12 [23] is higher than the Li-ion conductivity in NASICON-type Li 1.3 Al 0.3 Ti 1.7 (PO 4 ) 3 [25] , which implies that the Na-ion mobility in solid electrolytes is inherently higher than the Li ion mobility. This is because of the weaker Lewis acidity of Na ions, which have weaker electrostatic interaction with the oxide or sulfide anion species constituting the crystalline structure. However, Na-ion conducting sulfide electrolytes with the same degree of conductivity as that of the best Li ion conductor, LGPS, have not been discovered. Here we report a sulfide Na-ion conductor with ionic conductivity higher than the best Li-ion conductivity of 2.5 × 10 −2 S cm −1 in LGPS-type Li 9.54 Si 1.74 P 1.44 S 11.7 Cl 0.3 [4] . The sulfide superionic conductor with the composition of Na 2.88 Sb 0.88 W 0.12 S 4, obtained by replacing some of the antimony ions in Na 3 SbS 4 by aliovalent tungsten ions, exhibits a room temperature conductivity of 3.2 × 10 −2 S cm −1 in a sintered body; the conductivity is superior to those of any reported Li-ion and Na-ion conductors. In addition, the electrolyte shows good stability against hydrolysis, which is the origin of H 2 S gas evolution in an air atmosphere. The crystalline structure and electrical properties of Na 2.88 Sb 0.88 W 0.12 S 4 are also demonstrated and discussed. Material synthesis and structure analysis A mechanochemical process using a planetary ball mill apparatus was used to directly produce crystalline Na 3 SbS 4 (Supplementary Fig. 6a ), and its crystallinity increased after heat treatment at 275 °C for durations ranging from 1.5 to 12 h. X-ray diffraction (XRD) patterns of the Na 3− x Sb 1− x W x S 4 ( x = 0 and 0.12) electrolytes prepared by heat treatment are shown in Fig. 1a . The three Raman bands around 360, 380, and 410 cm −1 in the Raman spectrum (Fig. 1b ) of the prepared Na 2.88 Sb 0.88 W 0.12 S 4 reveals the presence of SbS 4 3− units, while the Raman band at ~470 cm −1 corresponds to the presence of WS 4 2− units, which are typically observed for crystalline Na 2 WS 4 . A fairly weak peak at ~420 cm −1 , probably due to WS 2 , is observed in the spectrum of Na 2.88 Sb 0.88 W 0.12 S 4 heated for 1.5 h, while no peak is observed for that heated for 12 h. The Raman bands of the other starting materials (Sb 2 S 3 , Na 2 S, S 8 ) are not observed in the spectra of Na 2.88 Sb 0.88 W 0.12 S 4 (Supplementary Fig. 1 ). Cross-section of the pelletized Na 2.88 Sb 0.88 W 0.12 S 4 heated at 275 °C for 12 h was observed by field-emission scanning electron microscopy (FE-SEM), and the secondary electron (SE) and backscattered electron (BSE) images are shown in Fig. 1c . As no composition-dependent contrast is observed in the BSE image, all the elements including tungsten are assumed to be uniformly dispersed in the monitored cross-section. In addition, energy-dispersive X-ray spectroscopic (EDX) mapping indicates the presence of tungsten in the entire SEM area (Supplementary Fig. 2 ). Elemental analysis using Rutherford backscattering spectrometry (RBS) predicts that the composition is Na 2.88 Sb 0.86 W 0.11 S 4 , and the error in the analysis of antimony is 0.86 ± 0.04. The experimentally determined composition is almost the same as the nominal composition of Na 2.88 Sb 0.88 W 0.12 S 4 . Fig. 1 Structural data for Na 3− x Sb 1− x W x S 4 ( x = 0 and 0.12) electrolytes prepared by heat treatment (H.T.) at 275 °C for 1.5–12 h. a X-ray diffraction patterns, b Raman spectra, and c cross-sectional SEM images (scale bar: 1 μm) of the prepared Na 3− x Sb 1− x W x S 4 Full size image Rietveld refinement analysis was conducted for the powder XRD pattern of the prepared Na 2.88 Sb 0.88 W 0.12 S 4 (Fig. 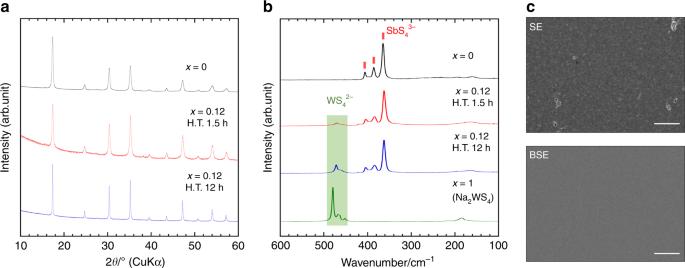Fig. 1 Structural data for Na3−xSb1−xWxS4(x= 0 and 0.12) electrolytes prepared by heat treatment (H.T.) at 275 °C for 1.5–12 h.aX-ray diffraction patterns,bRaman spectra, andccross-sectional SEM images (scale bar: 1 μm) of the prepared Na3−xSb1−xWxS4 2a ) and the results are shown in Supplementary Table 1 . Na 2.88 Sb 0.88 W 0.12 S 4 has a cubic structure ( a = 7.1920(1) Å, I- 43 m (no. 217), and the unit cell consists of a body-centered sublattice with SbS 4 3− and WS 4 2− units, and tungsten occupies the antimony site (2 a ), as shown in Fig. 2b . The W occupancy is 0.078(5), which is smaller than the W content at the nominal composition. The EDX and RBS results show that Sb is replaced by W based on the nominal composition. The W occupancy mismatch is believed to be based on the quality of XRD data measured using a laboratory X-ray diffractometer. Three-dimensional (3D) conduction of Na ions is expected in this cubic structure. The occupancy of the Na site (6 b ) is 0.974(2), suggesting the creation of vacancies in the lattice. The relatively large atomic displacement factor ( B ) of Na may be related to the dynamic motion of Na ions, as observed in the cubic Na 3 PS 4 phase [26] . Detailed structural analysis using synchrotron XRD is important to determine the W/Sb site occupancy and Na site vacancy in Na 2.88 Sb 0.88 W 0.12 S 4 . In contrast, Na 3 SbS 4 ( x = 0) has a tetragonal structure ( a = 7.1708(12) Å, c = 7.2376(2) Å, P- 42 1 c (no. 114)), which is in good agreement with the previous reports [11] , [12] ; The value of S obtained by the Rietveld refinement of Na 3 SbS 4 assuming a cubic phase was higher (i.e. S = R wp / R e = 3.34) than that ( S = 1.98) obtained assuming a tetragonal phase. Tetragonal Na 3 SbS 4 has two Na sites and their occupancies are unity, as shown in Supplementary Fig. 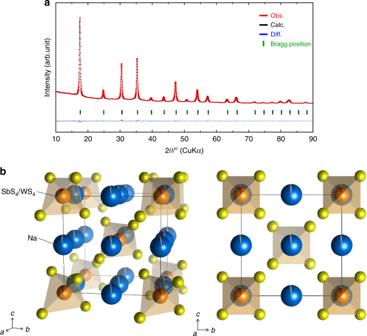Fig. 2 Crystal structure of Na2.88Sb0.88W0.12S4heated at 275 °C for 12 h.aRietveld refinement profiles of X-ray powder diffraction data for Na2.88Sb0.88W0.12S4. Red dots and black lines denote the observed and calculated XRD patterns, respectively. The green sticks mark the position of the reflections for Na2.88Sb0.88W0.12S4. The difference between the observed and calculated patterns is indicated by the blue line.bCrystal structure of cubic Na2.88Sb0.88W0.12S4with the unit cell outlined. The Na, Sb, W, and S sites are represented by blue, orange, gray, and yellow balls, respectively. Na is linearly arranged, and distortion of the Sb4/WS4tetrahedra is very small compared to the tetragonal structure of Na3SbS4(Supplementary Fig.3) 3 and Supplementary Table 2 . Na ion conduction along the c- axis in the tetragonal phase would be less likely than in the cubic phase [12] . It is noteworthy that the inclusion of tungsten into crystalline Na 3 SbS 4 is effective in introducing Na vacancies in the lattice, and it facilitates the formation of a cubic phase, which can facilitate isotropic 3D fast-ion conduction. Fig. 2 Crystal structure of Na 2.88 Sb 0.88 W 0.12 S 4 heated at 275 °C for 12 h. a Rietveld refinement profiles of X-ray powder diffraction data for Na 2.88 Sb 0.88 W 0.12 S 4 . Red dots and black lines denote the observed and calculated XRD patterns, respectively. The green sticks mark the position of the reflections for Na 2.88 Sb 0.88 W 0.12 S 4 . The difference between the observed and calculated patterns is indicated by the blue line. b Crystal structure of cubic Na 2.88 Sb 0.88 W 0.12 S 4 with the unit cell outlined. The Na, Sb, W, and S sites are represented by blue, orange, gray, and yellow balls, respectively. Na is linearly arranged, and distortion of the Sb 4 /WS 4 tetrahedra is very small compared to the tetragonal structure of Na 3 SbS 4 (Supplementary Fig. 3 ) Full size image Conduction characteristics Conductivity of the pelletized Na 2.88 Sb 0.88 W 0.12 S 4 was measured by the AC impedance method. Pellets of the material were prepared by cold-pressing the electrolyte powder at 1080 MPa, followed by heat treatment at 275 °C. 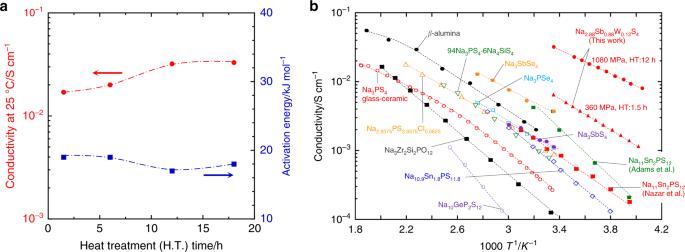Fig. 3 Conductive behavior of Na2.88Sb0.88W0.12S4electrolyte.aConductivity at 25 °C (σ25) and activation energyEafor the conduction of the pelletized Na2.88Sb0.88W0.12S4electrolytes as a function of heat treatment (H.T.) time at 275 °C. The pellets were prepared by cold-pressing the electrolyte powder at 1080 MPa, followed by heat treatment at 275 °C.bThe Arrhenius plot of the Na ion conductivity of the Na2.88Sb0.88W0.12S4electrolyte developed in this study and representative Na ion conductors reported so far 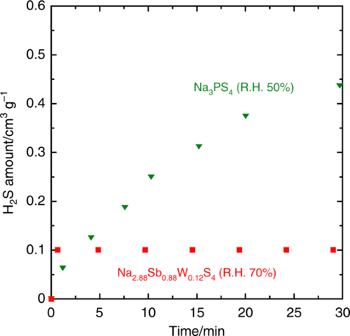Fig. 4 Monitoring H2S gas generated from Na2.88Sb0.88W0.12S4as a function of exposure time to humid air (relative humidity (R.H.) = 70%). The H2S content is normalized by the weight of sulfur in the samples. For comparison, the same measurement was carried out for Na3PS4under a less-humid condition of R.H. = 50% Figure 3a shows its conductivity at 25 °C ( σ 25 ) and activation energy E a for conduction as functions of the duration of heating at 275 °C. As an example, Nyquist plots at −25 °C for the pellets heated for 1.5 and 12 h are shown in Supplementary Fig. 4a , and the cross-sectional SEM image of the pellets are shown in Supplementary Fig. 4b . Only a spike owing to the capacitance at the interface between each electrolyte pellet and Au current collector is observed; other resistance components are not clearly detected in the high-frequency region even at a low measurement temperature of −25 °C. In this study, the total conductivity is thus determined from the resistance at the intersection of the spike and the x -axis; this resistance refers to the total resistance including both the grain-bulk and grain-boundary components of the electrolytes. Fig. 3 Conductive behavior of Na 2.88 Sb 0.88 W 0.12 S 4 electrolyte. a Conductivity at 25 °C ( σ 25 ) and activation energy E a for the conduction of the pelletized Na 2.88 Sb 0.88 W 0.12 S 4 electrolytes as a function of heat treatment (H.T.) time at 275 °C. The pellets were prepared by cold-pressing the electrolyte powder at 1080 MPa, followed by heat treatment at 275 °C. b The Arrhenius plot of the Na ion conductivity of the Na 2.88 Sb 0.88 W 0.12 S 4 electrolyte developed in this study and representative Na ion conductors reported so far Full size image The pellet heated for 1.5 h (relative density of 93%) has σ 25 of 1.7 × 10 −2 S cm −1 and E a of 19 kJ mol −1 . The electronic conductivity at 25 °C measured by a DC polarization technique is 7.9 × 10 −8 S cm −1 or lower, as shown in Supplementary Fig. 5 , which is five orders of magnitude lower than the total conductivity mentioned above; the Na-ion transport number of the prepared Na 2.88 Sb 0.88 W 0.12 S 4 is almost unity. Na-ion conductivity increased with an increase in the heating time as shown in Fig. 3a , because of the increase in the crystallinity of the cubic phase as well as the relative density of the pellet, as determined by the XRD analysis (Supplementary Fig. 6 ) and cross-sectional SEM imaging (Supplementary Fig. 4b ). The best conducting behavior is obtained for a pellet with a relative density of 95% obtained after heating for 12 h, which shows the highest σ 25 of 3.2 × 10 −2 S cm −1 and the lowest E a of 17 kJ mol −1 . Further, the conductivity of the material is definitely affected by the tungsten content ( x ) of Na 3− x Sb 1− x W x S 4 . Pellets of Na 3− x Sb 1− x W x S 4 with varying x were prepared by cold-pressing the milled Na 3− x Sb 1− x W x S 4 powders at 360 MPa, followed by heating at 275 °C for 1.5 h. XRD patterns of these pellets indicate the formation of cubic crystals without any impurity phases at all the compositions (Supplementary Fig. 7b ). No apparent peak shift in the XRD patterns is observed with increasing x . This is probably because of the nearly same ionic radii of Sb 5+ and W 6+ . The temperature-dependence of conductivities of the prepared pellets obeys the Arrhenius equation (Supplementary Fig. 6c ). The conductivity increases and the activation energy decreases with an increase in x , and better conductive behavior is achieved for x ranging from 0.12 to 0.15 (Supplementary Table 3 ). The electrolyte with x = 0.12 gives the lowest E a of 21 kJ mol −1 and a high conductivity of 6.4 × 10 −3 S cm −1 , which are superior to those of Na 3 SbS 4 ( x = 0) ( σ 25 of 2.1 × 10 −3 S cm −1 and E a of 26 kJ mol −1 ). Although this comparison is carried out among the lower density pellets prepared at a smaller molding pressure and a shorter heating time, the partial substitution of tungsten for antimony definitely improves the Na-ion conductivity of the Na 3 SbS 4 electrolyte. The Arrhenius plot of the Na-ion conductivity of the Na 2.88 Sb 0.88 W 0.12 S 4 electrolyte developed in this study is shown in Fig. 3b ; it shows the highest conductivity among Na-ion conductors reported so far. In addition, σ 25 of 3.2 × 10 −2 S cm −1 for the electrolyte is higher than that of the best LGPS-type Li 9.54 Si 1.74 P 1.44 S 11.7 Cl 0.3 Li-ion conductor ( σ 25 = 2.5 × 10 −2 S cm −1 ). Here, we have successfully discovered for the first time, a Na-ion-conducting sulfide electrolyte that has higher conductivity than all known Li-ion conductors. Exposure to the atmosphere Another advantage of the Na 2.88 Sb 0.88 W 0.12 S 4 electrolyte is its high tolerance to air; that is, the amount of harmful H 2 S generated when it is exposed to air is almost negligible. H 2 S generation from the electrolyte even under a highly humid environment (relative humidity, R.H. of 70%) is suppressed when compared to that from a conventional Na 3 PS 4 under a less-humid condition with R.H. of 50% (Fig. 4 ). An XRD pattern similar to that of the hydrate, Na 3 SbS 4 ·9H 2 O is observed for the electrolyte after exposure to humid air (Supplementary Fig. 8 ). The formation of a hydrate compound without H 2 S generation has already been reported for crystalline Na 3 SbS 4 [11] ; our tungsten-substituted sulfide conductor also undergoes a similar structural transformation with hydration. Fig. 4 Monitoring H 2 S gas generated from Na 2.88 Sb 0.88 W 0.12 S 4 as a function of exposure time to humid air (relative humidity (R.H.) = 70%). The H 2 S content is normalized by the weight of sulfur in the samples. For comparison, the same measurement was carried out for Na 3 PS 4 under a less-humid condition of R.H. = 50% Full size image In conclusion, a Na 2.88 Sb 0.88 W 0.12 S 4 superionic conductor was developed. The conductivity of this material, 3.2 × 10 −2 S cm −1 is the highest among sulfide Li and Na-ion conductors reported so far. The generation of Na vacancies and stabilization of the cubic phase by the partial substitution of antimony in Na 3 SbS 4 with tungsten are responsible for its superior conduction. The Na 2.88 Sb 0.88 W 0.12 S 4 electrolyte with high tolerance to H 2 S gas generation under an ambient atmosphere would improve safety of all-solid-state batteries and reduce manufacturing cost. The developed sulfide superionic conductor contributes to the realization of solid-state batteries with high-energy density and power density. Material synthesis Na 3− x Sb 1− x W x S 4 solid electrolytes were prepared via a mechanochemical process using a planetary ball mill apparatus (Pulverisette 7, Fritsch GmbH). Reagent-grade Na 2 S (Nagao Co., 99.1%), Sb 2 S 3 (Nihonseiko Co., 99.8%), WS 2 (Aldrich Chem. Co., 99%), and S (Aldrich Chem. Co., 99.98%) powders were used as the starting materials. The starting materials were weighed at stoichiometric compositions of Na 3− x Sb 1− x W x S 4 (e.g., the molar ratio of Na 2 S:Sb 2 S 3 :S = 50.0:16.7:33.3 for Na 3 SbS 4 and the molar ratio of Na 2 S:Sb 2 S 3 :S:WS 2 = 48.0:14.7:33.3:4 for Na 2.88 Sb 0.88 W 0.12 S 4 ). A mixture of the starting materials (0.6 g) was ground using a mortar and a pestle for 10 min and placed in a 45 mL ZrO 2 pot containing 250 ZrO 2 balls of diameter 4 mm. Then, the starting materials were milled at a rotation speed of 510 rpm for 5 or 30 h. It was further subjected to heat treatment at 275 °C for several hours (1.5–18 h) in a porcelain crucible to obtain the final Na 3− x Sb 1− x W x S 4 electrolytes. The colors of the prepared electrolytes Na 3 SbS 4 and Na 2.88 Sb 0.88 W 0.12 S 4 were brown and dark brown, respectively. All the steps were carried out in dry Ar atmosphere. Material characterization The crystallographic phase was identified using an X-ray diffractometer (SmartLab, Rigaku) with Cu- Kα radiation. Diffraction data were collected in steps of 0.02° in the 2 θ range 10−60° at a scan rate of 10° min −1 . X-ray diffraction (XRD) measurements were performed using an airtight vessel with a beryllium window to prevent the sample from exposure to air. The crystalline structure was refined using the computer program PDXL2 (Rigaku Co.), and the crystal models were visualized using the VESTA software [27] . Rietveld refinement was performed for the XRD data collected in steps of 0.02° in the 2 θ range 10−120° at a scan rate of 2° min −1 . For this, first, the peak shape, background coefficient, scale factor, and lattice constants were refined. Then, the occupancy was fixed at the stoichiometric composition, and the atomic displacement factor was refined. Finally, the above parameters were fixed, and the occupancy, except for sulfur, was refined. Raman spectroscopy was carried out on a Raman spectrophotometer (LabRAM HR-800, Horiba) equipped with a 532 nm He–Ne laser to identify the structural units. The electrolyte samples were placed in an airtight vessel filled with dry Ar gas, and Raman scattering signals from the samples were collected through a transparent quartz plate mounted on the upper side of the vessel. Scanning electron microscopy was carried out on a FE-SEM (SU8220, Hitachi High-Technologies) equipped with an energy-dispersive X-ray spectroscopy system (EDX, EMAXEvolution X-MAX, Horiba Ltd.). The samples were transferred from an airtight vessel with dry Ar gas to the apparatus. The chemical composition was determined by RBS. The RBS measurement was carried out with He + beam accelerated to 2.3 MeV using customized RC-43 (National Electrostatics Co.). The sample was set in a high-vacuum chamber with the sample surface perpendicular to the ion beam. The beam current was measured with a Faraday cup and then tuned to 10 nA. Energy spectrum of the backscattered He + was obtained using a surface barrier detector (SBD) set at 160°. The alpha rays emitted from the sample due to nuclear reactions were also detected with an SBD set at 146°. The RBS spectrum was collected for ~2 h under the measurement condition. The RBS revealed that the ball-milled sample contained about 0.06 wt% of Zr. The amount is, however, so less that the influence of Zr contamination from the ball-milling media on the properties of Na 2.88 Sb 0.88 W 0.12 S 4 is almost negligible. The amounts of H 2 S gas evolved from Na 2.88 Sb 0.88 W 0.12 S 4 were measured using a H 2 S gas sensor (GBL-HS, JIKCO Co.) and a humidity controller (SCS01, I.E. Service Co.). The H 2 S gas evolved from Na 3 PS 4 was also measured for comparison. A powder-compressed pellet (100 mg) was placed in a 2-L sealed container, where the air humidity and temperature were controlled to 70% and 24–26 °C, respectively. The amount of H 2 S was normalized by the mass of sulfur in the samples. Electrical characterization The ionic conductivity of pelletized Na 2.88 Sb 0.88 W 0.12 S 4 electrolytes was measured by the AC impedance method. The data were collected in the range of 10Hz–1M Hz using an impedance analyzer (1260, Solartron) with an applied AC voltage of 10–25 mV. The milled samples were cold pressed at 360 or 1080 MPa into pellets and then heated at 275 °C for several hours to obtain the final electrolyte pellets. The diameter and thickness of the pellets were 10 and ~1 mm, respectively. Gold current collectors were used to cover the entire surface of both sides of the pellet. The pellet was sealed in a laminate-type pouch cell to prevent air exposure. The conductivity was measured in the temperature range of ca. −25 to 25 °C, controlled with an ethanol-cooled bath and a constant temperature bath. As an example, three specimens of Na 2.88 Sb 0.88 W 0.12 S 4 prepared by pressing at 360 MPa and heating at 275 °C for 1.5 h showed almost the same conductivities ranging from 6.4 × 10 −3 to 6.7 × 10 −3 S cm −1 at 25 °C (Supplementary Table 3 ). The activation energy for conduction was calculated from the slope of the Arrhenius equation, σ = σ 0 exp(− E a / RT ), where σ is the ionic conductivity, T is the absolute temperature, σ 0 is the pre-exponential factor for ionic conduction, E a is the activation energy for the ionic conduction, and R is the gas constant. The errors in activation energy can be considered to be small, because the R 2 values (coefficient of determination) for the Arrhenius plots exceed 0.99. The electronic conductivity was measured on electrolyte pellet samples via a DC polarization technique. The data were collected using a potentio/galvanostat (1287, Solartron) with the applied DC voltages ranging from 0.07 to 0.98 V at 25 °C.